A platform for designing hyperpolarized magnetic resonance chemical probes Hyperpolarization is a highly promising technique for improving the sensitivity of magnetic resonance chemical probes. Here we report [ 15 N, D 9 ]trimethylphenylammonium as a platform for designing a variety of hyperpolarized magnetic resonance chemical probes. The platform structure shows a remarkably long 15 N spin–lattice relaxation value (816 s, 14.1 T) for retaining its hyperpolarized spin state. The extended lifetime enables the detection of the hyperpolarized 15 N signal of the platform for several tens of minutes and thus overcomes the intrinsic short analysis time of hyperpolarized probes. Versatility of the platform is demonstrated by applying it to three types of hyperpolarized chemical probes: one each for sensing calcium ions, reactive oxygen species (hydrogen peroxide) and enzyme activity (carboxyl esterase). All of the designed probes achieve high sensitivity with rapid reactions and chemical shift changes, which are sufficient to allow sensitive and real-time monitoring of target molecules by 15 N magnetic resonance. Considerable effort has long been dedicated to the molecular analysis of living systems. In particular, molecular analysis has recently been attempted for complex systems in cell assembly, tissue, organ and body. Magnetic resonance (MR)-based techniques—MR imaging (MRI) or MR spectroscopy—are the powerful approaches for such in situ molecular analysis, and various MR chemical probes (MR probes) have been designed [1] . However, these have an intrinsic limitation for practical applications, namely their low sensitivity. Hyperpolarization is a highly promising technique for overcoming this limitation [2] , [3] . The hyperpolarization technique achieves polarization of nuclear spin populations, producing a large enhancement of sensitivity for MR-detectable nuclei. The technique has been applied successfully for in vitro or in vivo metabolic analyses using stable isotope-enriched natural compounds (metabolites), including N -acetylated amino acids, pyruvate, fructose, choline and glucose [4] , [5] , [6] , [7] , [8] . It was recently demonstrated that the hyperpolarization technique can also be applied to chemical sensors for surveying the chemical status of living systems. In practice, hyperpolarized [ 13 C]bicarbonate [9] , [ 13 C]benzoylformic acid [10] , [ 13 C, D 6 ] p -anisidine [11] and [ 13 C]dehydroascorbate [12] , [13] have been designed as sensitive MR probes for sensing pH, H 2 O 2 , HOCl and redox status, respectively. A universal strategy—in other words, the presence of a platform structure for designing hyperpolarized MR probes—can make it easier to develop a variety of hyperpolarized MR sensors. The importance of a platform structure is obvious, as demonstrated in the design of optical probes. For example, in the case of fluorescent probes, some chromophores work as a platform [14] . A good representative is fluorescein ( Fig. 1a ). A variety of fluorescent probes have been developed from this fluorophore platform using a well-established strategy ( vide infra ). However, corresponding structures for hyperpolarized MR probes have not yet been realized. 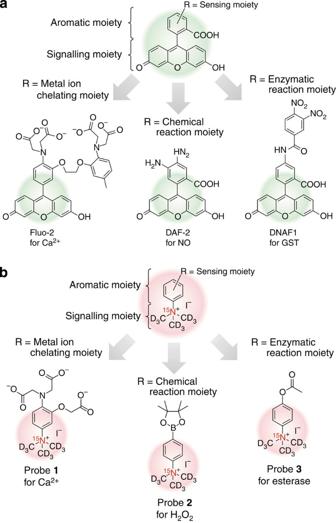Figure 1: Platform for designing chemical probes. (a) Fluorescein as a platform for designing fluorescent probes. Fluorescein comprises both aromatic and signalling moieties. The fluorescence quantum yield of the signalling moiety can be tuned by the highest occupied molecular orbital (HOMO)/lowest unoccupied molecular orbital (LUMO) level of the aromatic moiety. In three examples—Fluo-2, DAF-2 and DNAF1—the HOMO/LUMO level of the aromatic moiety is changed on the binding or reaction of Ca2+, NO and glutathioneS-transferase enzyme with the sensing moiety, respectively, leading to light emission from the fluorescent sensors. (b) Proposed platform for designing hyperpolarized MR probes. Various hyperpolarized MR probes can be designed by the same strategy used for converting fluorophore platforms to fluorescent sensors, as shown inFig. 1a. The chemical structures of probes1–3used in this study are shown. Figure 1: Platform for designing chemical probes. ( a ) Fluorescein as a platform for designing fluorescent probes. Fluorescein comprises both aromatic and signalling moieties. The fluorescence quantum yield of the signalling moiety can be tuned by the highest occupied molecular orbital (HOMO)/lowest unoccupied molecular orbital (LUMO) level of the aromatic moiety. In three examples—Fluo-2, DAF-2 and DNAF1—the HOMO/LUMO level of the aromatic moiety is changed on the binding or reaction of Ca 2+ , NO and glutathione S -transferase enzyme with the sensing moiety, respectively, leading to light emission from the fluorescent sensors. ( b ) Proposed platform for designing hyperpolarized MR probes. Various hyperpolarized MR probes can be designed by the same strategy used for converting fluorophore platforms to fluorescent sensors, as shown in Fig. 1a . The chemical structures of probes 1 – 3 used in this study are shown. Full size image Here we propose [ 15 N, D 9 ]trimethylphenylammonium ([ 15 N, D 9 ]TMPA) as a promising platform structure for designing hyperpolarized MR probes. It achieves improved sensitivity with a remarkably long hyperpolarization lifetime ( 15 N, T 1 =816 s, 14.1 T). The versatile applicability of the platform structure is established by designing three types of hyperpolarized MR probes, one each targeting metal ion (Ca 2+ ), reactive oxygen species (H 2 O 2 ), and enzyme (carboxyl esterase). Design of platform structure for hyperpolarized MR probes Typically, a platform structure in an optical imaging probe is composed of signalling, aromatic and sensing moieties ( Fig. 1 ), where the aromatic unit works as a connector to transmit chemical events on a sensing moiety (R in Fig. 1 ) to a signalling moiety [15] , [16] . In the case of fluorescein, benzoic acid and xanthene chromophore act as the aromatic and signalling moieties, respectively ( Fig. 1a ). Derivatization of benzoic acid (the aromatic moiety) with sensing moieties enables the generation of various signal-on-type fluorescent probes, for example, Fluo-2 for Ca 2+ [17] , DAF-2 for NO [18] and DNAF1 for glutathione S -transferase (GST) sensing [19] . In the present case, the signalling moieties are MR-detectable hyperpolarized nuclei ( Fig. 1b ). When attempting to design a platform for hyperpolarized MR probes, one critical issue is the short lifetime of the hyperpolarized spin state of the nuclei (signalling moieties). For example, the hyperpolarization lifetime of a 13 C MR probe is only a few tens of seconds at best, which restricts its application to the analysis of extremely fast kinetic events. Therefore, the challenge is to find a hyperpolarized nucleus or structure that affords a much longer hyperpolarization lifetime. The hyperpolarization lifetime is related directly to the spin–lattice relaxation time ( T 1 ) [20] . The T 1 of 15 N nuclei in organic compounds is usually longer than those of 1 H and 13 C nuclei [21] . In addition, this spin–lattice relaxation is caused mainly by dipole–dipole interaction, spin–rotation interaction and chemical shift anisotropy [22] , [23] , [24] . Therefore, typically, 15 N nuclei, which have less neighbouring protons in small and rigid structures tend to give a longer T 1 value, achieving a longer hyperpolarization lifetime. Actually, the 15 N nucleus of choline ( 15 N(CH 3 ) 3 CH 2 CH 2 OH) has been shown to produce a long hyperpolarization lifetime [7] . With this in mind, we designed [ 15 N]trimethylphenylammonium ([ 15 N]TMPA or [ 15 N]trimethylaniline) as a candidate for the platform structure ( Fig. 1b ). We anticipated that [ 15 N]TMPA, which has a – 15 N(CH 3 ) 3 signalling moiety on an aromatic moiety, might serve as a suitable platform for designing hyperpolarized MR probes. Long hyperpolarization lifetime of the platform structure The [ 15 N]TMPA was synthesized from [ 15 N]aniline by nucleophilic displacement with CH 3 I. The hyperpolarization lifetime of [ 15 N]TMPA was evaluated by measuring the T 1 value ( Fig. 2a ). The 15 N T 1 value of [ 15 N]TMPA was determined as 275±11 s (14.1 T, D 2 O, 30 °C), which was much longer than that of the practically used [1- 13 C]pyruvic acid (41 s, 14.1 T, D 2 O, 30 °C). Interestingly, this value is longer than that of [ 15 N]choline (232 s, 14.1 T, D 2 O, 30 °C). Reduced interaction with proton (less dipole–dipole interaction) or structural rigidity (less spin–rotation interaction) might explain this longer T 1 value [22] , [23] , [24] . 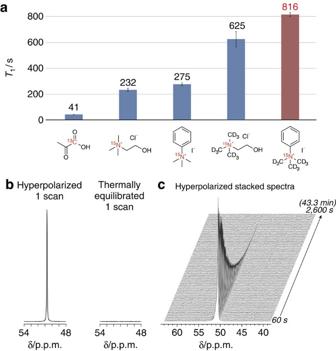Figure 2: Properties of proposed platform [15N, D9]TMPA. (a) Spin–lattice relaxation timeT1(14.1 T, D2O, 30 °C) of13C (450 mM) or15N (200–300 mM) nuclei of the chemical compound shown at the bottom. Error bars indicate a s.d. of five saturation recovery measurements. (b) Single-scan15N NMR spectra of hyperpolarized (40 s after dissolution) or thermally equilibrated [15N, D9]TMPA (10 mM). (c) Single-scan15N NMR spectra of hyperpolarized [15N, D9]TMPA stacked from ca. 60–2,600 s (every 20 s, 128 times) after dissolution of the hyperpolarized [15N, D9]TMPA (5 mM). The pulse angles for15N measurements inbandcwere 90° and 13°, respectively. Figure 2: Properties of proposed platform [ 15 N, D 9 ]TMPA. ( a ) Spin–lattice relaxation time T 1 (14.1 T, D 2 O, 30 °C) of 13 C (450 mM) or 15 N (200–300 mM) nuclei of the chemical compound shown at the bottom. Error bars indicate a s.d. of five saturation recovery measurements. ( b ) Single-scan 15 N NMR spectra of hyperpolarized (40 s after dissolution) or thermally equilibrated [ 15 N, D 9 ]TMPA (10 mM). ( c ) Single-scan 15 N NMR spectra of hyperpolarized [ 15 N, D 9 ]TMPA stacked from ca. 60–2,600 s (every 20 s, 128 times) after dissolution of the hyperpolarized [ 15 N, D 9 ]TMPA (5 mM). The pulse angles for 15 N measurements in b and c were 90° and 13°, respectively. Full size image The T 1 value was further extended by deuteration of [ 15 N]TMPA. Non-proton-coupled nuclei tend to show a longer T 1 value because of the lack of dipole–dipole interactions with neighbouring protons. In this sense, deuteration is one of the most straightforward ways to increase the hyperpolarization lifetime [25] , [26] , [27] , [28] . We prepared [ 15 N, D 9 ]TMPA, wherein all the methyl protons were replaced with deuterium atoms using CD 3 I instead of CH 3 I. As a result, the [ 15 N, D 9 ]TMPA afforded a remarkably long 15 N T 1 value of 816±15 s (14.1 T, D 2 O, 30 °C; 754±23 s in 90% H 2 O; Fig. 2a ), which was 19.9-, 3.5- and 1.3-fold longer than those of [1- 13 C]pyruvic acid, [ 15 N]choline and [ 15 N, D 9 ]choline, respectively. To the best of our knowledge, this T 1 value is the longest among the 15 N compounds reported to date. The [ 15 N, D 9 ]TMPA was efficiently hyperpolarized by dynamic nuclear polarization (DNP) using trityl radicals [29] . The sensitivity of the hyperpolarized sample increased and allowed detection of the targeted 15 N by a single scan (% P 15N =2.0%, T =298 K, B 0 =9.4 T, 1.5 h polarization). The high sensitivity was obvious when compared with the thermally equilibrated spectrum ( Fig. 2b ). As little as 10 μM of hyperpolarized [ 15 N, D 9 ]TMPA could be detected (S/N ratio=3) using a single-scan 15 N analysis under our experimental conditions (flip angle=90°). In addition, because of its remarkably long T 1 value, the hyperpolarized state continued after dissolution of the hyperpolarized sample (stacked spectra; Fig. 2c ). These results indicate that deuterated [ 15 N, D 9 ]TMPA has a considerable potential for use as a remarkably long-lived and sensitive hyperpolarization unit. Hyperpolarized MR probe targeting calcium ions With the [ 15 N, D 9 ]TMPA platform in hand, we then demonstrated its practical utility by designing new hyperpolarized MR probes. These needed to satisfy the following prerequisites: (1) the probe should have a MR-detectable nucleus with a long T 1 for long hyperpolarization; (2) it should bind/react with the target species rapidly within the hyperpolarization lifetime; and (3) it should induce a sufficiently large chemical shift change upon reaction. As a first choice, we aimed to develop the hyperpolarized MR probe targeting the calcium ion (Ca 2+ ), a biologically important metal ion [30] . In addition to their biological importance, abnormal Ca 2+ concentrations in the blood (hyper- or hypocalcemia) are known to be associated with some diseases [31] , [32] ; therefore, the in situ analysis and imaging of Ca 2+ concentrations in the body is potentially useful for an investigation of the mechanism or an early diagnosis of these diseases. We designed MR probe 1 ( Fig. 3a ), wherein the [ 15 N, D 9 ]TMPA (aromatic and signalling moieties) has been substituted with triacetic acid as a Ca 2+ -chelating group (sensing moiety) [33] . MR probe 1 was synthesized from the methyl ester of o -aminophenol- N , N , O -triacetic acid (APTRA), a known Ca 2+ chelator, in four steps ( Supplementary Methods ). The absorption analyses confirmed that probe 1 bound to Ca 2+ rapidly with an affinity of K d =490 μM ( Supplementary Fig. S1a,d ), with one-to-one binding stoichiometry ( Supplementary Fig. S1b,c ) and high selectivity over Mg 2+ or K + ( Supplementary Fig. S1e ). 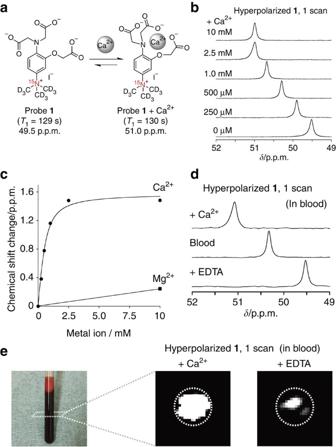Figure 3: Hyperpolarized MR probe targeting calcium ions. (a) Ca2+sensing by MR probe1. (b) Single-scan15N NMR spectra of hyperpolarized probe1(0.5 mM) with various concentrations of Ca2+in HEPES pH 7.4 (40 s after mixing, 30° pulse angle). (c) Plot of15N chemical shift change of hyperpolarized probe1(0.5 mM) versus concentrations of Ca2+(circles) and Mg2+(square). (d) Single-scan15N NMR spectra (30° pulse angle) of hyperpolarized probe1(0.5 mM) in human blood containing 50% v/v HEPES buffer (middle) without or (top) with 10 mM Ca2+or (bottom) with 10 mM EDTA. (e) Single-scan15N MRI image of hyperpolarized probe1(8 mM) in HEPES buffer containing 20% v/v human blood with (left) 8 mM of Ca2+or (right) 8 mM of EDTA. The photograph of Ca2+-added sample is shown in left. Figure 3: Hyperpolarized MR probe targeting calcium ions. ( a ) Ca 2+ sensing by MR probe 1 . ( b ) Single-scan 15 N NMR spectra of hyperpolarized probe 1 (0.5 mM) with various concentrations of Ca 2+ in HEPES pH 7.4 (40 s after mixing, 30° pulse angle). ( c ) Plot of 15 N chemical shift change of hyperpolarized probe 1 (0.5 mM) versus concentrations of Ca 2+ (circles) and Mg 2+ (square). ( d ) Single-scan 15 N NMR spectra (30° pulse angle) of hyperpolarized probe 1 (0.5 mM) in human blood containing 50% v/v HEPES buffer (middle) without or (top) with 10 mM Ca 2+ or (bottom) with 10 mM EDTA. ( e ) Single-scan 15 N MRI image of hyperpolarized probe 1 (8 mM) in HEPES buffer containing 20% v/v human blood with (left) 8 mM of Ca 2+ or (right) 8 mM of EDTA. The photograph of Ca 2+ -added sample is shown in left. Full size image The sensitivity of MR probe 1 was enhanced dramatically by DNP. As expected, the 15 N of MR probe 1 had a long T 1 value (129±22 s, 9.4 T) and the hyperpolarized state of 15 N signal was observed by 15 N single-scan nuclear magnetic resonance (NMR; 600 s under our experimental conditions, 10 mM of 1 , Supplementary Fig. S2 ). The hyperpolarized MR probe 1 worked as a chemical shift-switching Ca 2+ sensor. Figure 3b shows the single-scan 15 N NMR spectra of hyperpolarized MR probe 1 (0.5 mM) in the presence of various concentrations of Ca 2+ (0–10 mM). The presence of Ca 2+ induced a 15 N chemical shift change (from 49.5 to 51.0 p.p.m. ; Δ δ =~1.5 p.p.m.) in a Ca 2+ concentration-dependent manner, which was sufficient to be detected by 15 N DNP–NMR analysis ( Fig. 3b,c ). In marked contrast, only a small chemical shift change ( δ =0.3 p.p.m.) was observed in the presence of excess Mg 2+ (10 mM) ( Fig. 3c ). Importantly, the hyperpolarized Ca 2+ probe worked in biological samples. In blood serum, T 1 value of MR probe 1 was not shortened (142±2 s, 9.4 T, in blood serum containing 50% v/v D 2 O). Thus, 15 N signals of hyperpolarized MR probe 1 (0.5 mM) were detectable in human blood ( Fig. 3d ). The observed signal could be discriminated clearly from those in blood samples with a Ca 2+ excess (10 mM Ca 2+ , added externally, top spectrum) and a Ca 2+ deficiency (10 mM EDTA, added externally, bottom spectrum). Estimated from a calibration curve in human serum ( Supplementary Fig. S3 ), the observed 15 N signal in blood corresponded to 1.04 mM of Ca 2+ (typical total Ca concentration in blood (50% v/v)=1~1.25 mM). This value was close to that (1.15 mM) determined using a classical optical sensing method for Ca 2+ . The small difference between the results from MR and optical analyses might be caused by a difference of protocols. In the case of the optical sensing of Ca 2+ concentration in blood, a purification step is indispensable because the inherent light absorption by blood interferes with the optical measurements, as shown in Fig. 3e (left). In fact, we prepared blood plasma by centrifugation and used it for optical Ca 2+ sensing. On the other hand, hyperpolarized MR analysis can be carried out in blood directly. This in situ (in blood) applicability is an advantage of the present calcium-sensing MR probe. To show the applicability of the hyperpolarized MR probe 1 , we applied probe 1 for Ca 2+ imaging in blood ( Fig. 3e ). The 15 N signal of the probe 1 +Ca 2+ complex was imaged ( Fig. 3e ). An image with good contrast was obtained in blood samples with a Ca 2+ excess (8 mM Ca 2+ , added externally, left image), whereas weak contrast was observed in blood with a Ca 2+ deficiency (8 mM EDTA, added externally, right image). These results indicate that the hyperpolarized MR probe 1 works as an in situ Ca 2+ sensor with high sensitivity even in human blood. Versatility of the platform The versatility of the platform was confirmed by designing two other hyperpolarized MR probes targeting different molecules but by the same strategy. Probe 2 was designed as a hyperpolarized MR probe targeting H 2 O 2 ( Fig. 4a ), which is one of major disease-related reactive oxygen species [34] , [35] . H 2 O 2 production is associated with endothelial inflammatory responses [35] and the increased production level of H 2 O 2 in tumours is correlated with cancer cell growth and malignancy [36] . The probe has an H 2 O 2 -reactive boronic acid ester (the sensing moiety) on the [ 15 N, D 9 ]TMPA unit ( Supplementary Methods ) [37] . After reaction with H 2 O 2 , the boronic acid was expected to convert to a hydroxyl group and such functional group transformation would induce a chemical shift change of the hyperpolarized 15 N to function as a chemical shift-switching MR probe. This proved to be the case. The T 1 values of probe 2 and product 2 were determined as 444±11 and 486±66 s (9.4 T), respectively, which were sufficiently long to be monitored by 15 N DNP–NMR spectroscopy. The apparent reaction kinetics were very rapid at (4.8±0.4) × 10 –3 s –1 ( Supplementary Fig. S4 ). As shown in the single-scan 15 N NMR spectra of Fig. 4b , a new signal of product 2 (49.3 p.p.m.) was observed from single-scan after starting the 15 N NMR measurement (corresponding to 50 s after mixing the hyperpolarized probe 2 with 0–6.18 mM of H 2 O 2 ). Because of almost the same T 1 values of probe and product—that is, almost the same decay rate of hyperpolarized spin state—the signal ratio of the hyperpolarized product to the amount of probe and product was proportional to the concentration of H 2 O 2 ( Fig. 4b ), displaying a good linear correlation with increasing concentrations ( Fig. 4c ). 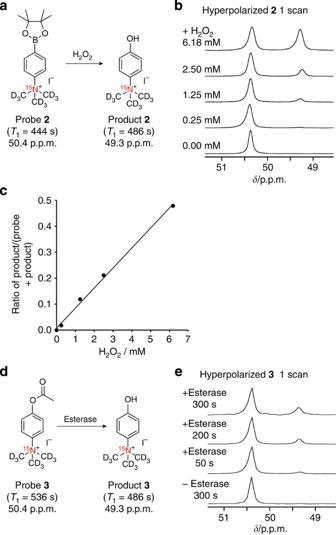Figure 4: Hyperpolarized MR probes targeting hydrogen peroxide and carboxyl esterase. (a) H2O2sensing by MR probe2. (b) Single-scan15N NMR spectra of hyperpolarized probe2(2.5 mM) mixed with various concentrations (0, 0.25, 1.25, 2.50 and 6.18 mM) of H2O2in phosphate buffer pH 7.4 (50 s after mixing, 30° pulse angle). (c) Plot of product2/(probe2+product2) peak integral ratios versus concentrations of H2O2,R2=0.996 for linear fitting. (d) Esterase activity sensing by MR probe3. (e) Single-scan15N NMR spectra of hyperpolarized probe3(10 mM, 15° pulse angle) after mixing with esterase (124 units ml−1, derived from the porcine liver) in PBS (pH 7.4). Figure 4: Hyperpolarized MR probes targeting hydrogen peroxide and carboxyl esterase. ( a ) H 2 O 2 sensing by MR probe 2 . ( b ) Single-scan 15 N NMR spectra of hyperpolarized probe 2 (2.5 mM) mixed with various concentrations (0, 0.25, 1.25, 2.50 and 6.18 mM) of H 2 O 2 in phosphate buffer pH 7.4 (50 s after mixing, 30° pulse angle). ( c ) Plot of product 2 /(probe 2 +product 2 ) peak integral ratios versus concentrations of H 2 O 2 , R 2 =0.996 for linear fitting. ( d ) Esterase activity sensing by MR probe 3 . ( e ) Single-scan 15 N NMR spectra of hyperpolarized probe 3 (10 mM, 15° pulse angle) after mixing with esterase (124 units ml −1 , derived from the porcine liver) in PBS (pH 7.4). Full size image In addition, the platform was applied successfully in designing a hyperpolarized MR probe for analysing carboxyl esterase activity. The carboxyl esterase is a biomarker of cancer [38] and one of the major enzymes related to drug metabolism and pro-drug activation [39] . For example, human carboxyl esterase 2 is commonly expressed in tumour tissues and is correlated with the activation of anticancer drugs [40] . Therefore, detection of carboxyl esterase is biologically and medically significant. Probe 3 , with a methyl ester moiety, was designed ( Supplementary Methods ) as a hyperpolarized MR probe for esterase ( Fig. 4d ) and incubated with a model carboxyl esterase derived from porcine liver. As with probes 1 and 2 , probe 3 also showed a long T 1 value (536±33 s for the probe and 486±66 s for its product at 9.4 T), sufficient enhancement of signal intensity and 15 N chemical shift change (1.1 p.p.m.) after reaction with esterase. A new 15 N signal of product 3 (49.3 p.p.m.) appeared in the presence of carboxyl esterase ( Fig. 4e ), in addition to the parent peak of probe 3 (50.4 p.p.m.). This allowed us to detect the presence of carboxyl esterase from the hyperpolarized 15 N chemical shift analysis. We propose [ 15 N, D 9 ]TMPA as a suitable platform for designing various hyperpolarized MR probes. The significance of this study can be summarized as follows. First is the proposed platform’s high performance. The [ 15 N, D 9 ]TMPA platform achieved good hyperpolarization and a remarkably long hyperpolarization lifetime with the longest T 1 value (816 s, 14.1 T, D 2 O) among the 15 N compounds reported to date. This extended lifetime enabled the detection of the hyperpolarized 15 N signal of the platform for several tens of minutes under our experimental conditions, approaching the lifetimes of molecular probes used for positron emission tomography [41] . This overcomes the intrinsic short analysis time of hyperpolarized probes. Given that existing hyperpolarized chemical probes (typically 13 C-based) have much shorter T 1 values (≤60 s), this long-lived hyperpolarized chemical probe is useful because it allows easy handling, sufficient distribution through the body and long duration measurements of targeted biological events. In addition, the longer hyperpolarization can lower the probe concentration required. This is a distinct advantage of the present platform. The second important aspect of this platform is its ease of incorporation into sensors. It comprises signalling (hyperpolarized 15 N) and aromatic (benzene ring) moieties. The platform can be converted to a hyperpolarized 15 N MR probe by the same strategy used for designing fluorescent sensors ( Fig. 1a ), that is, by the simple derivatization of an aromatic moiety with an appropriate sensing moiety. As various fluorescent probes have already been designed using this strategy, the [ 15 N, D 9 ]TMPA platform has high potential to be diversified to create hyperpolarized MR sensors targeting various biochemical events. The third advantage of [ 15 N, D 9 ]TMPA is its versatility. Three different types of hyperpolarized MR probes were designed successfully from the same platform ( Fig. 1b ). All of the designed compounds worked as sensitive, selective and fast responsive hyperpolarized MR probes. Further, it was demonstrated that the designed hyperpolarized MR sensor could be utilized for 15 N MRI of target biomolecules in blood. These findings demonstrate the considerable potential of [ 15 N, D 9 ]TMPA as a basis for designing a variety of hyperpolarized MR probes. Although the present research showed the high potential of the platform for generating hyperpolarized MR probes, there are still aspects to be improved. Practical in vivo applications of these probes must await further studies on biostability, toxicity and distribution. However, as demonstrated for fluorescent probes, these factors could be overcome by making improvements to the probes or the platform itself. In fact, preliminary experiments showed that the cytotoxicity and inhibitory activity against acetylcholine esterase could be suppressed markedly by appropriate substitutions to the TMPA platform (probes 1 and 3 showed almost no cytotoxicity at the low mM range, Supplementary Fig. S5 ). In addition, efforts should be made towards development of a clinical 15 N scanner, optimized for the hyperpolarized 15 N sensor. General information on synthesis Reagents and solvents were purchased from standard suppliers and used without further purification. Gel permeation chromatography (GPC) was performed on JAIGEL GS310 using a JAI Recycling Preparative HPLC LC-9201. NMR spectra were measured using a Bruker Avance III spectrometer (400 MHz for 1 H). Methanol-d 4 (3.31 p.p.m.) or D 2 O (4.79 p.p.m.) was used as the internal standard for 1 H NMR. Methanol-d 4 (49.0 p.p.m.) and methanol in D 2 O (49.5 p.p.m.) were used as the internal standard for 13 C NMR. Choline chloride- 15 N (43.4 p.p.m.) was used as the external standard for 15 N NMR. Mass spectra were measured using a JEOL JMS-HX110A fast atom bombardment (FAB). Synthesis of [ 15 N, D 9 ]choline chloride Potassium carbonate (4.46 g, 32.3 mmol) and [D 3 ]iodomethane (3.12 g, 21.5 mmol) were added to [ 15 N]ethanolamine (334 mg, 5.38 mmol) in dry methanol (15 ml), and the mixture was stirred under nitrogen atmosphere at room temperature for 12 h. After insoluble inorganic salt was removed by filtration, the filtrate was evaporated under reduced pressure. The residue was mixed with small amount of dry methanol, filtered and the filtrate was evaporated. The residue was washed with ethyl acetate:methanol=10:1 and the remaining solid was collected to give [ 15 N, D 9 ]choline iodide as a pale yellow solid (741 mg, 59%): 1 H NMR (CD 3 OD, 400 MHz) δ =3.60–3.63 (m, 2H), 4.04–4.07 (m, 2H); 13 C NMR (CD 3 OD, 100 MHz) δ =55.8, 67.4; 15 N NMR (CD 3 OD, 40 MHz) δ =43.8. Silver oxide (1.53 g, 6.59 mmol) was added to [ 15 N, D 9 ]choline iodide (741 mg, 3.19 mmol) in dry methanol (10 ml) and the mixture was stirred for 30 min. Solids were removed by filtration. HCl aqueous solution (0.5 M) was added dropwise to the filtrate until pH became 4 and then the solvent was evaporated under reduced pressure. Dry ethanol (10 ml) was added to the residue and insoluble solids were removed by filtration. The solvent was evaporated under reduced pressure from the filtrate to give [ 15 N, D 9 ]choline chloride as a pale yellow solid (147 mg, 31%). 1 H NMR (D 2 O, 400 MHz) δ =3.42–3.44 (m, 2H), 3.96–4.00 (m, 2H); 13 C NMR (D 2 O, 100 MHz) δ=53.1–54.0 (m), 56.2, 67.7; 15 N NMR (D 2 O, 40 MHz) δ =43.1; HRMS (FAB): m/z calc. for C 5 H 5 D 9 O 15 N + [M−Cl] + =114.1611, found=114.1611. Synthesis of [ 15 N]TMPA Iodomethane (330 μl, 5.30 mmol) was added to a solution of [ 15 N]aniline (100 mg, 1.06 mmol) and N,N -diisopropylethylamine (740 μl, 4.25 mmol) in dry dimethylformamide (3 ml). The mixture was stirred at room temperature overnight and evaporated under vacuum. Ethyl acetate was added to the residue resulting in a white precipitate. The resulting precipitate was filtered and purified using GPC (eluent: methanol) to give [ 15 N]TMPA as a white powder (105 mg, 37%): 1 H NMR (CD 3 OD, 400 MHz) δ =3.73 (d, J =0.8 Hz, 9 H), 7.61–7.70 (m, 3H), 7.96–7.99 (m, 2H); 13 C NMR (CD 3 OD, 100 MHz) δ =56.6 (d, J =5 Hz), 119.8 (d, J =1 Hz), 130.3, 130.3 (d, J =1 Hz), 147.2 (d, J =8 Hz); 15 N NMR (CD 3 OD, 40 MHz) δ =53.3; HRMS (FAB): m/z calc. for C 9 H 14 15 N + [M−I] + =137.1097, found=137.1098. Synthesis of [ 15 N, D 9 ]TMPA [D 3 ]Iodomethane (622 μl, 10.0 mmol) was added to a solution of [ 15 N]aniline (188 mg, 2.00 mmol) and N,N -diisopropylethylamine (1.39 ml, 8.00 mmol) in dry dimethylformamide (3 ml). The mixture was stirred at room temperature overnight and then at 50 °C overnight. After evaporation under vacuum, ethyl acetate was added to the residue resulting in a white precipitate. The resulting precipitate was filtered and purified using GPC (eluent: methanol) to give [ 15 N, D 9 ]TMPA as a white powder (375 mg, 69%): 1 H NMR (CD 3 OD, 400 MHz) δ =7.62–7.71 (m, 3H), 8.01–8.04 (m, 2H); 13 C NMR (CD 3 OD, 100 MHz) δ =119.9 (d, J =1 Hz), 130.3, 130.3 (d, J =1 Hz), 147.0 (d, J =8 Hz); 15 N NMR (CD 3 OD, 40 MHz) δ =52.3; HRMS (FAB): m/z calc. for C 9 H 5 D 9 15 N + [M−I] + =146.1662, found=146.1665. T 1 measurements All T 1 measurements were performed at thermally equilibrated conditions. The T 1 measurements in Fig. 2a were performed using a JEOL ECA 600 (14.1 T, 30 °C) by the saturation recovery method. The T 1 measurements of MR probes 1 , 2 , 3 ( Figs 3 and 4 ) were performed using a Bruker Avance III spectrometer (9.4 T, 25 °C) by the inversion recovery method. General information on DNP–NMR/MRI measurements Tris{8-carboxyl-2,2,6,6-tetra[2-(1-hydroxyethyl)]-benzo(1,2-d:4,5-d′)bis(1,3)dithiole-4-yl}methyl sodium salt (Ox63 radical, GE Healthcare) and the 15 N-labelled sample were dissolved in a 1:1 solution of D 2 O (99.9%, D):dimethyl sulfoxide-d6 (99.8%, D; final concentration of Ox63 15 mM). The sample was submerged in liquid helium in a DNP polarizer magnet (3.35 T; HyperSense, Oxford Instruments). The transfer of polarization from the electron spin on the radical to the 15 N nuclear spin on the probe was achieved using microwave irradiation at 94 GHz and 100 mW for 1.5 or 3.0 h under 2.8 mbar at 1.4 K. After polarization, samples were dissolved in water containing 0.025% EDTA disodium salt or an appropriate buffer heated to 10 bar. The DNP–NMR measurements of Figs 2b , 3 , and were performed using JEOL ECA 300 (7.05 T). The DNP–NMR measurement of Fig. 2c was performed using Japan Redox JXI-400Z spectrometer (9.4 T). Choline chloride- 15 N (43.4 p.p.m.) was used as the external standard for 15 N NMR. The DNP–NMR spectra were obtained using flip angles of 13° ( Fig. 2c ), 15° ( Fig. 4e ), 23° ( Supplementary Fig. S2 ), 30° ( Figs 3b–d and 4b ) or 90° ( Fig. 2b ). The DNP–MRI measurement of Fig. 3e was performed using Varian 400 MR WB spectrometer (9.4 T). 15 N DNP–NMR (time course analysis of [ 15 N, D 9 ]TMPA) The hyperpolarized [ 15 N, D 9 ]TMPA (final concentration 5 mM) was dissolved in water containing 0.025% EDTA disodium salt (6 ml). The solution was passed through an anion exchange cartridge (Grace) to remove the remaining Ox63 radical, which affects the hyperpolarization lifetime, and then transferred to a 10-mm NMR tube. 15 N DNP–NMR (Ca 2+ sensing by probe 1 ) The hyperpolarized probe 1 (final concentration 0.5 mM) was dissolved in various concentrations of Ca 2+ (final concentrations: 0, 0.25, 0.5, 1.0, 2.5 or 10 mM) or Mg 2+ (final concentration: 10 mM) in 20 mM HEPES buffer (pH 7.4, 4 ml), and then an aliquot was transferred to a 5-mm NMR tube. 15 N DNP–NMR (Ca 2+ sensing by probe 1 in human blood) The hyperpolarized probe 1 (final concentration 0.5 mM) dissolved in 20 mM HEPES buffer (pH 7.4, 1 ml) was added to human blood (1 ml) with or without externally added Ca 2+ or EDTA (final concentrations: 10 mM) and an aliquot was transferred to a 5-mm NMR tube. 15 N DNP–MRI (Ca 2+ sensing by probe 1 in human blood) The hyperpolarized probe 1 (final concentration: 8 mM) was dissolved in 20 mM HEPES buffer (pH 7.4, 4 ml) with Ca 2+ (final concentration: 8 mM) or EDTA-2Na (final concentration: 8 mM). The solution was added to human blood (1 ml) in a 10-mm NMR tube and mixed. DNP–MRI images were acquired with a gradient echo two-dimensional multi-slice acquisition technique (GEMS) with a total acquisition time of 0.64 ms. The excitation pulse was centred at probe 1 +Ca 2+ complex. Other MR parameters were field of view 40 × 40 mm 2 × 4 mm, matrix size of 32 × 32, 60° radio frequency pulse. In the reconstruction phase, the matrix was zero-filled to 64 × 64. 15 N DNP–NMR (H 2 O 2 sensing by probe 2 ) The hyperpolarized probe 2 (final concentration: 2.5 mM) dissolved in phosphate buffer (pH 7.4, 3.9 ml) was mixed with various concentrations of H 2 O 2 (final concentration: 0–6.18 mM, 100 μl) and an aliquot was transferred to a 5-mm NMR tube. The concentration of H 2 O 2 was determined based on the molar extinction coefficient at 240 nm (43.6 M –1 cm –1 ). 15 N DNP–NMR (esterase sensing by probe 3 ) The hyperpolarized probe 3 (500 μl, final concentration: 10 mM) dissolved in PBS (pH 7.4) was mixed with esterase (Sigma-Aldrich E2884, 62 units, 8 μl) and transferred to a 5-mm NMR tube. The esterase was derived from the porcine liver, which was used as a model esterase. How to cite this article: Nonaka, H. et al. A platform for designing hyperpolarized magnetic resonance chemical probes. Nat. Commun. 4:2411 doi: 10.1038/ncomms3411 (2013).